Repeated targeting of the same hosts by a brood parasite compromises host egg rejection Cuckoo eggs famously mimic those of their foster parents to evade rejection from discriminating hosts. Here we test whether parasites benefit by repeatedly parasitizing the same host nest. This should make accurate rejection decisions harder, regardless of the mechanism that hosts use to identify foreign eggs. Here we find strong support for this prediction in the African tawny-flanked prinia ( Prinia subflava ), the most common host of the cuckoo finch ( Anomalospiza imberbis ). We show experimentally that hosts reject eggs that differ from an internal template, but crucially, as the proportion of foreign eggs increases, hosts are less likely to reject them and require greater differences in appearance to do so. Repeated parasitism by the same cuckoo finch female is common in host nests and likely to be an adaptation to increase the probability of host acceptance. Thus, repeated parasitism interacts with egg mimicry to exploit cognitive and sensory limitations in host defences. Avian brood parasites lay their eggs in other birds’ nests, leaving all parental care to the host [1] . They are ideal to investigate sensory and cognitive mechanisms underlying decision-making because visual information is pivotal to their interactions. Information leads to a reduction in uncertainty about an aspect of the environment or current state [2] and is crucial in making effective choices [3] . However, greater uncertainty exists when sources of information are ambiguous or mechanisms underlying decision-making are conflicting, and antagonists such as parasites could exploit this to their own advantage. Many host species reject foreign eggs, resulting in the evolution of egg mimicry by parasites. Hosts are more likely to reject eggs that differ more from their own in perceptual terms [4] , [5] , [6] , [7] , [8] . However, to reject a parasitic egg successfully, hosts must also identify which eggs are theirs and which are a parasite’s. To do so, hosts could either use a simple rule of thumb and reject the odd one out in a clutch (the ‘discordancy hypothesis’) or reject eggs that differ from a learnt or innate (inherited) internal template of their own egg appearance (‘true recognition’) [9] , [10] , [11] . Most work supports the template-based hypothesis [12] , [13] , [14] , [15] , [16] , although discordancy mechanisms exist in some species [17] , [18] and may occur alongside template (true) recognition [19] , [20] . Regardless of the mechanisms, the two key problems that hosts must solve are to discriminate between eggs (a sensory task) and to recognize their own eggs (a cognitive task). An antagonist, such as a parasite, would benefit from exploiting either or both of these processes. Despite widespread evidence that hosts generally reject eggs that differ from an internal template, such a mechanism should have significant sources of error. First, maintenance of memory is costly and imperfect [21] , and a memorized template need not precisely match a host’s current eggs. Second, eggs differ in appearance within and between clutches, and according to viewing angle and light conditions, and learning itself may be constrained by variability in the host’s eggs [10] . Such sources of uncertainty could hinder successful decision-making. Likewise, when parasitized nests contain two or more foreign eggs and host eggs are not in the majority, rejection by discordancy may result in hosts rejecting their own eggs. Combining template and discordancy mechanisms could partly overcome their respective limitations [19] because hosts could compare each egg to their template and to the proportion of eggs that match it sufficiently well. However, as host eggs become increasingly outnumbered, eggs that sufficiently match the host’s (imperfect) template become fewer, allowing fewer comparisons between the eggs in the nest and the host’s template. Therefore, as the ratio of parasitic to host eggs increases we predict that the incidence of host rejection should be less likely and requires greater phenotypic differences, because only large differences will give reliable information about which eggs are foreign. Repeated parasitism may exploit such weaknesses in host defences by creating conflicting information. We tested these predictions in the tawny-flanked prinia and its parasite, the cuckoo finch. Egg appearance (colour and pattern) varies greatly among individuals in both host and parasite, but individual females always lay a single egg-type throughout their lives [7] , [8] . Cuckoo finches do not target prinia clutches that resemble their own eggs but instead rely on chance matches to succeed [7] . Therefore, mimicry can range from very good to poor. A cuckoo finch female commonly lays two eggs in the same host nest [22] (see below). Here, we show that prinias prioritize a template-based approach to identify foreign eggs, but that they also utilize information about the relative proportions of their own and foreign eggs in making rejection decisions. Second, we show that hosts are less likely to reject foreign eggs when they outnumber their own and when the level of mimicry is very good, and correspondingly cuckoo finch eggs are more likely to be accepted under such circumstances. Finally, we show that cuckoo finch females have a strategy of repeatedly targeting the same host nests with more than one egg to increase the likelihood of acceptance, and this constitutes a further adaptation by brood parasites to defeat host defences. Hosts reject eggs based on a template-matching mechanism We first determined whether hosts reject foreign eggs using discordancy or a template-based mechanism. As with previous experiments investigating egg rejection in cuckoo finch hosts [7] , [8] , we swapped conspecific prinia eggs (of approximately the same stage of incubation) between clutches and monitored which eggs were rejected. We presented hosts with eggs that differed from their own to varying degrees and ensured that these included experimental clutches involving well-matched experimental eggs, so as to generate some difficult discrimination tasks [7] . Unlike our previous experiments, in which we replaced one egg per nest, we swapped sets of eggs between nests to generate rejection trials with ratios of host to experimental eggs of 2:2 ( n =11), 1:2 ( n =33) and 1:3 ( n =4) ( Fig. 1 ). If hosts use discordancy in rejection, then they should reject their own eggs when outnumbered by foreign eggs, whereas if hosts use template recognition, then they should reject the foreign eggs regardless of their proportion in the clutch [13] . In 17 trials all eggs were accepted, whereas in 31 trials hosts rejected one or more eggs. In 25 trials hosts rejected all experimental eggs, leaving only their own (even when outnumbered by 1:2 or 1:3; Fig. 2 ). In three cases, hosts rejected one of the two experimental eggs. On only three occasions did hosts reject one of their own eggs, and in all three cases the colour match (the most important predictor of rejection [7] ) was very good (2.3, 2.2 and 3.4 discrimination units or ‘just noticeable differences’ (JNDs); Fig. 2 and Methods). Therefore, hosts were significantly more likely to reject foreign eggs than their own (binomial test: P <0.001). 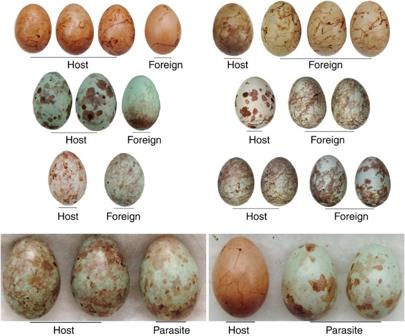Figure 1: Examples of experimental clutches and naturally parasitized nests. The top images show the range of colours and patterns found in prinia eggs, and the proportions of host and foreign eggs used in rejection trials (ratios of host:foreign eggs). Lines under the eggs indicate groups originating from the same clutch. The bottom two images show naturally parasitized clutches with one cuckoo finch egg (left) or two cuckoo finch eggs (right). Both cuckoo finch and host eggs show extensive variation among individuals. Prinia eggs have fine lines on them that cuckoo finches do not reproduce; surprisingly, hosts do not seem to use this fail-safe ‘signature’ in egg rejection decisions. Such markings make it easy to distinguish host and parasite eggs. Average host egg size for length is 15.63 mm (max=16.98, min=14.63) and breadth is 11.42 mm (max=11.91, min=10.82) from a sample of 40 randomly chosen eggs. Figure 1: Examples of experimental clutches and naturally parasitized nests. The top images show the range of colours and patterns found in prinia eggs, and the proportions of host and foreign eggs used in rejection trials (ratios of host:foreign eggs). Lines under the eggs indicate groups originating from the same clutch. The bottom two images show naturally parasitized clutches with one cuckoo finch egg (left) or two cuckoo finch eggs (right). Both cuckoo finch and host eggs show extensive variation among individuals. Prinia eggs have fine lines on them that cuckoo finches do not reproduce; surprisingly, hosts do not seem to use this fail-safe ‘signature’ in egg rejection decisions. Such markings make it easy to distinguish host and parasite eggs. Average host egg size for length is 15.63 mm (max=16.98, min=14.63) and breadth is 11.42 mm (max=11.91, min=10.82) from a sample of 40 randomly chosen eggs. 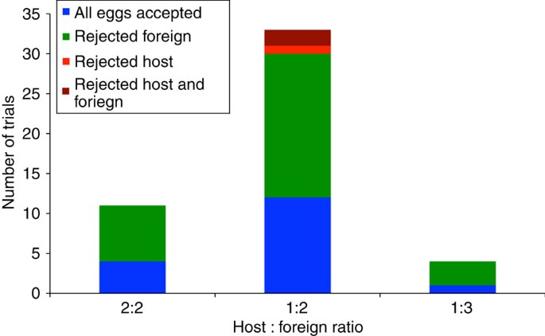Figure 2: Host behaviour in relation to the proportion of foreign eggs. In 31 of 48 trials hosts showed rejection behaviour, but in only three of these did they reject any of their own eggs: in two trials hosts rejected one experimental and one host egg, and in one trial they rejected only a host egg. Full size image Figure 2: Host behaviour in relation to the proportion of foreign eggs. In 31 of 48 trials hosts showed rejection behaviour, but in only three of these did they reject any of their own eggs: in two trials hosts rejected one experimental and one host egg, and in one trial they rejected only a host egg. Full size image The proportion of foreign eggs affects host rejection Next, we tested whether rejection probability depended on the degree of mimicry and the proportion of foreign eggs present. We combined the egg rejection experiments above (excluding the three trials where hosts rejected one of their own eggs, and one trial where we did not have both colour and pattern information) with our previously published [7] rejection trials where we swapped just one host egg between clutches, but otherwise used identical methods. This gave trials involving ratios of host to foreign eggs of 3:1 ( n =33), 2:1 ( n =76), 1:1 ( n =16), 2:2 ( n =10), 1:2 ( n =30) and 1:3 ( n =4). Of these 169 trials, 79 involved acceptances and 90 involved rejections. We then used colour and pattern analyses to calculate discrepancies in each aspect of egg appearance, allowing us to determine which factor predicted egg rejection. We quantified the difference between host and foreign eggs as perceived by bird colour and luminance vision (measured in discrimination units), and for five aspects of egg pattern: marking size, dispersion, contrast, diversity and proportion coverage [23] , [24] (Methods). We modelled the predictors of egg rejection using generalized linear models with a binomial error structure. Reported P -values are based on the final model that was selected based on Akaike information criterion (AIC) weightings. Significant predictors of egg rejection were: marking diversity ( P =0.008), marking size ( P =0.004), proportion of experimental eggs ( P =0.018) and the interaction between proportion of experimental eggs and colour difference ( P =0.029). Additional nonsignificant terms retained in the selected model were colour ( P =0.465), luminance ( P =0.119), marking dispersion ( P =0.124) and contrast ( P =0.149). The significant interaction between proportion of experimental eggs and colour difference revealed that as the proportion of foreign eggs increases, hosts are less likely to reject them and require larger differences in colour to do so ( Fig. 3 ). 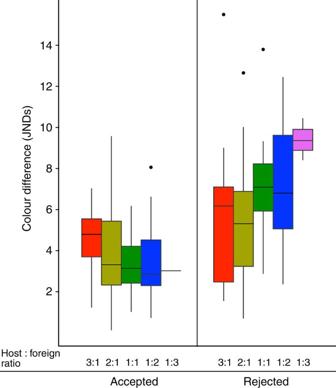Figure 3: Host behaviour in relation to the proportion of foreign eggs and the level of colour difference between eggs. Foreign eggs were more likely to be rejected the more they differed in colour from the host’s own eggs. However, this effect was dependent on their relative proportions in the nest. As foreign eggs increased in number, hosts required a greater difference in colour to reject them. Colour differences are discrimination units or ‘just noticeable differences’ (JNDs), where a JND of <1.0 means that two objects cannot be discriminated, and values between 1.00 and 3.00 should be difficult to discriminate. Boxplots show median bars and interquartile ranges; whiskers show outer quartiles. There were 79 trials with eggs accepted and 90 trials with eggs rejected (see Results). Figure 3: Host behaviour in relation to the proportion of foreign eggs and the level of colour difference between eggs. Foreign eggs were more likely to be rejected the more they differed in colour from the host’s own eggs. However, this effect was dependent on their relative proportions in the nest. As foreign eggs increased in number, hosts required a greater difference in colour to reject them. Colour differences are discrimination units or ‘just noticeable differences’ (JNDs), where a JND of <1.0 means that two objects cannot be discriminated, and values between 1.00 and 3.00 should be difficult to discriminate. Boxplots show median bars and interquartile ranges; whiskers show outer quartiles. There were 79 trials with eggs accepted and 90 trials with eggs rejected (see Results). Full size image Cuckoo finches benefit from repeated parasitism Finally, we conducted simulation modelling to determine the likelihood of real cuckoo finch eggs being accepted or rejected by hosts in nests with different proportions of host and parasitic eggs. Following our previous approach [8] , we calculated the difference in egg appearance between 999 randomly chosen pairs of prinia ( n =300) and cuckoo finch ( n =84) eggs from our study population. Colour and pattern differences for each pair were substituted into the experimental model to provide the predicted z -value attributed to each pairing using the ‘predict’ function in R, from which the rejection likelihood was produced by a reverse-logit calculation. Simulations were repeated for all combinations of host:parasite egg ratios. Thus, our model of real prinia egg rejection could be used to calculate how well real cuckoo finch eggs would have fared in different prinia nests [8] with clutches comprising different ratios of host to parasitic eggs. The simulations showed that cuckoo finch eggs are less likely to be rejected when they comprise a greater proportion of the host clutch ( Fig. 4a ). This effect is particularly pronounced when colour mimicry is good: for example, eggs very similar to the hosts’ (up to two JNDs difference) have a rejection probability (upper and lower 95% confidence interval (CI)) of 0.64 (0.89, 0.29) when there is a host:parasite egg ratio of 3:1, but a rejection probability of 0.09 (0.45, 0.01) when there is a host:parasite egg ratio of 1:2 ( Fig. 4b ). Such relatively close matches in colour are likely to be common: of the 999 host–parasite comparisons, 24% of pairs have colour differences of <5 JNDs (approximately where the lines for different egg ratios converge in Fig. 4b ). 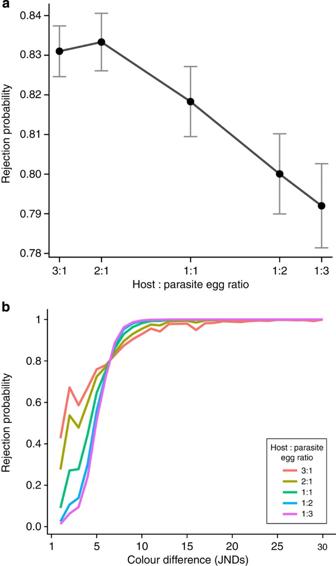Figure 4:Probability of rejection of real cuckoo finch eggs with different host:parasite egg ratios. (a) Simulations between 999 random pairs of host and cuckoo finch eggs show that as the proportion of parasitic eggs in the nest increases, they are more likely to be accepted. Error bars show ±1 s.e.m. (b) The probability of rejection also depends on the level of colour difference between host and parasitic eggs: closely matching eggs are less likely to be rejected when they comprise a greater proportion of the clutch. Figure 4: Probability of rejection of real cuckoo finch eggs with different host:parasite egg ratios . ( a ) Simulations between 999 random pairs of host and cuckoo finch eggs show that as the proportion of parasitic eggs in the nest increases, they are more likely to be accepted. Error bars show ±1 s.e.m. ( b ) The probability of rejection also depends on the level of colour difference between host and parasitic eggs: closely matching eggs are less likely to be rejected when they comprise a greater proportion of the clutch. Full size image Naturally parasitized clutches at our study site during 2007–2009 and 2012–2013 are consistent with the prediction that repeated parasitism should benefit the cuckoo finch: of 62 parasitized prinia nests where the final clutch composition was known (that is, incubation had begun), two-thirds contained either two (61%) or three (5%) parasitic eggs laid by the same female (as assessed phenotypically by the human eye; cuckoo finch eggs are highly variable and distinctive among individuals for colour and pattern [7] , making it relatively easy to identify eggs as belonging to the same individuals). Parasitic eggs were in the majority in 68% of nests (in 36 of 42 cases, no host eggs were present), equal numbers of host and parasitic eggs were present in 19% of nests, and host eggs made up the majority of the clutch in just 13% of parasitized nests. Avian brood parasites have evolved a suite of adaptations to facilitate access to host nests and acceptance of their young, including mimicry at the egg, chick, fledgling and adult stages [5] , [7] , [12] , [25] , [26] , [27] . The coevolutionary battleground of the egg stage poses two main challenges for host parents. First, they must detect that a foreign egg is present in the nest, which requires them to discriminate between their own eggs and those of a parasite (a sensory task). Second, they must reject the correct egg(s), which requires them to recognize correctly which eggs belong to each party (a cognitive task). For a parasite to be successful, it must defeat either or both these defences. In this study, we demonstrate a novel evolutionary tactic at play in these interactions. We have previously shown that the tawny-flanked prinia, the most common host of the cuckoo finch, uses several different features of egg colour and pattern to discriminate between its eggs and those of the cuckoo finch. In this study, we first demonstrated that prinias know the appearance of their own eggs and primarily reject foreign eggs based on whether they deviate from this internal template. This is consistent with past work investigating mechanisms of rejection in hosts of other brood parasites [11] , [12] , [13] , [14] , [16] , [20] . However, we further demonstrated that prinias do not simply reject any eggs that differ sufficiently from an internal template regardless of their frequency. Instead, they appear to use both template-recognition and discordancy mechanisms to maximize information about egg identity. The two mechanisms are in conflict when host eggs are outnumbered by mimetic parasitic eggs, such that sensory and cognitive mechanisms disagree. We have shown that under such circumstances, hosts prioritize information from the template-recognition mechanism but require greater colour differences to make the correct decision. This conflict of information can be exploited by a parasitic strategy of repeated laying in the same host nest, such that a parasitic female’s eggs outnumber the host’s own. A simulation model based on our field experimental data demonstrated that a parasite’s eggs are more likely to be accepted if she lays more than one egg in the same host nest, especially when the level of mimicry is also good. This implies a strong adaptive benefit to observed cuckoo finch behaviour: the majority of naturally parasitized nests in the field are composed of clutches in which cuckoo finch eggs are either equal in number to or outnumber host eggs. Such repeated targeting of the same nest is unlikely to be explained by a shortage of hosts, as tawny-flanked prinias are abundant at the study site and parasitism levels are only ~ 19% (ref. 7 ). Our simulations suggest that approximately a quarter of cuckoo finch breeding attempts have levels of mimicry that afford a benefit from repeated parasitism. Are any costs of repeated parasitism likely to mitigate these benefits of increased host acceptance? In the common cuckoo ( Cuculus canorus ), previous work has shown that multiple parasitism increases the likelihood of egg acceptance by some hosts [28] as a greater number of foreign eggs lead to reduced rejection behaviour, perhaps due to similar conflict between mechanisms and uncertainty as we have shown here [19] . However, cuckoo chicks eject all other nest occupants such that only one parasite ever survives to fledge, and cuckoo eggs in the same nest are accordingly laid by different females [28] . Furthermore, in populations where multiple parasitism occurs, overall parasitism rates are very high and it is likely that multiple parasitism results from parasite population size relative to host density, rather than any counter-adaptation to beat host defences. This contrasts with the repeated parasitism by the individual females observed in cuckoo finches. Cuckoo finch chicks do not actively kill their nest-mates [22] , and hosts often successfully rear broods of two parasitic chicks [22] : for 13 prinia nests where we followed cuckoo finch nestlings to within a week of fledging, 11 nests (85%) contained two parasitic chicks and just two nests contained a single parasite. Hence, cuckoo finches should gain a net benefit from repeatedly targeting the same host nest. We conclude that in complex natural systems such as host–parasite coevolution, the use of sensory information in discrimination can interact with cognitive mechanisms to control decision-making, and uncertainty in these mechanisms can be exploited by antagonists such as parasites or competitors. Rejection experiments Rejection experiments (undertaken with permission from the Zambia Wildlife Authority) were conducted in ~ 800 ha on and around Musumanene Farm (16 o 47′S, 26 o 54′E), Zambia, during January–March 2007–2009 by C.N.S. [7] and 2012 by M.S., J.T. and C.N.S. Each trial involved a different female, replacing one or more eggs from the clutch with the equivalent number of eggs from another clutch. Nests were monitored daily, where possible, for 3–4 days unless rejection or predation occurred earlier. Eggs missing from the nest were considered rejected. Rejection almost always occurred by day 3 (ref. 7 ). Quantification of egg appearance and mimicry Analysis of egg pattern and colour followed previous approaches [7] , [8] , [24] . Using reflectance spectra taken with Ocean Optics USB2000 and USB4000 spectrometers and irradiance spectra from host nests [7] , we calculated photon catches for a blue tit’s ( Cyanistes caeruleus ) single and double cones [29] . These were used in a log form of a discrimination model [30] that predicts colour and luminance discrimination to yield JNDs, where discrimination is unlikely with values <3. Five aspects of egg pattern were obtained from digital image analysis, in which we Fourier-transformed the images and then used bandpass filtering to analyse the information (energy) at different spatial frequencies (scales) [24] . This yielded measures of marking size, contrast, variability, pattern proportion (the proportion of the egg surface covered with markings) and dispersion (the difference in coverage between the egg’s two poles). Absolute differences between host and experimental/parasitic eggs were taken for each pattern measurement. We used one egg per clutch for the colour and pattern measurements, which are repeatable within clutches [7] , [8] . Parasitic egg data came from the same site in the same years as the experiments. Statistical modelling Differences between host and experimental egg colour, luminance, volume, five pattern variables and incubation state and year were included in the statistical model (performed in R ref. 31 ). An interaction with the proportion of experimental eggs in the clutch was included for all terms. The final model was selected using stepwise addition and subtraction of terms based on Akaike information criterion [32] and explained 44.0% of variance in the incidence of rejection behaviour [33] . How to cite this article: Stevens, M. et al. Repeated targeting of the same hosts by a brood parasite compromises host-egg rejection. Nat. Commun. 4:2475 doi: 10.1038/ncomms3475 (2013).